Unexpected interplay of bonding height and energy level alignment at heteromolecular hybrid interfaces Although geometric and electronic properties of any physical or chemical system are always mutually coupled by the rules of quantum mechanics, counterintuitive coincidences between the two are sometimes observed. The coadsorption of the organic molecules 3,4,9,10-perylene tetracarboxylic dianhydride and copper-II-phthalocyanine on Ag(111) represents such a case, since geometric and electronic structures appear to be decoupled: one molecule moves away from the substrate while its electronic structure indicates a stronger chemical interaction, and vice versa for the other. Our comprehensive experimental and ab-initio theoretical study reveals that, mediated by the metal surface, both species mutually amplify their charge-donating and -accepting characters, respectively. This resolves the apparent paradox, and demonstrates with exceptional clarity how geometric and electronic bonding parameters are intertwined at metal–organic interfaces. In chemistry, there is a general tendency that stronger bonds go along with shorter bond lengths. For covalent bonds, this is well known; for instance, in the sequence from single to triple bonds, the bond length decreases while the bond strength increases. Shorter bonding distances imply more wave function overlap, stronger hybridization and (in case of polar bonds) more charge exchange, all of which promote stronger chemical interaction and can thus be interpreted as electronic signatures thereof. Therefore, it would be very surprising if observations which would normally go along with a stronger chemical interaction coincide with a larger bonding distance. Yet, such a counterintuitive relationship is precisely what we observe in the particular case of a metal–organic hybrid interface presented here. For adsorbed organic molecules, the relevant geometric parameter (the ‘bond length’) is the vertical adsorption height above the metal. Hence, one would expect that a smaller adsorption height should correspond to stronger chemical interaction. Indeed, it was recurrently observed that on more reactive surfaces, where chemical interaction is stronger, the adsorption heights tend to be smaller [1] , [2] , [3] , [4] , [5] , [6] , [7] , [8] , [9] , [10] , [11] , [12] . This empirical correlation is often a result of both local and extended (that is, π-) bonds [12] and of the charge spill-out profile above the surface (see below). In the electronic structure an observation that usually goes along with smaller adsorption height and thus stronger chemical interaction is a downshift of the lowest unoccupied molecular orbital (LUMO), that is, an increase of its binding energy. In the case of ‘weak chemisorption’, which is the relevant situation for the molecule–substrate combination discussed in this paper, this includes an at least partially filling of the LUMO, which hence becomes detectable in photoelectron spectroscopy. Two effects are at the origin of this relationship between adsorption height and LUMO binding energy. First, the work function of the metal controls both adsorption height and LUMO binding energy: if the work function is low, the spatial extent of the charge spill out is small. This favours both small adsorption heights [5] , [12] , [13] , [14] and—assuming vacuum level alignment—large LUMO binding energies. Note that the push-back effect, that is, the Pauli repulsion of the electronic charge spill out of the metal caused by the approaching molecule, even strengthens this correlation: a larger push-back tends to reduce adsorption height and work function further, yielding even larger orbital binding energies. Second, the interaction of the negatively charged LUMO with its image dipole increases the LUMO binding energy, the more so the closer the molecule is to the surface. The normal relationship between geometric and electronic structure for molecules adsorbing on metal surfaces therefore is the following: a smaller bonding distance, which is the geometric signature of a stronger chemical interaction, coincides with a increased binding energy of the relevant frontier orbital (here: the LUMO). This relationship has been demonstrated for many organic materials. Two examples are the aromatic molecules copper-II-phthalocyanine (CuPc) and 3,4,9,10-perylene tetracarboxylic dianhydride (PTCDA). Their adsorption on noble metal surfaces (Ag, Cu and Au) has been investigated intensively within the last years [3] , [9] , [10] , [14] , [15] , [16] , [17] , [18] , [19] , [20] , [21] , [22] , [23] , [24] , [25] , [26] , [27] . Here we focus on the adsorption of these two molecules on the Ag(111) surface, where both molecules exhibit weak chemisorption [28] , [29] . The adsorption behaviour of both molecules exhibits some characteristic differences: the charge transfer from the surface to the molecule is stronger for PTCDA than for CuPc, which agrees with the adsorption heights found for both adsorbate systems. Furthermore, while PTCDA molecules on Ag(111) attract each other and hence form compact islands in the submonolayer regime ( Fig. 1a ) [30] , CuPc (and other phthalocyanine) molecules repel each other on Ag(111) and thus yield a dilute phase ( Fig. 1b ) and a low-density phase with a continuously changing unit cell size as function of coverage [3] , [25] , [31] . This remarkable disparity emerges from a different interplay between intermolecular and molecule–substrate interactions in the two homomolecular systems. While a repulsive intermolecular force is present in both systems due to the molecule–surface bond dipole, this is exceeded by the attractive interaction between the quadrupole moments of neighbouring PTCDA molecules. It is therefore interesting to examine whether a mixed, heteromolecular phase between the two can be prepared, and how the differences in the intermolecular and molecule–substrate interactions affect the geometric and electronic properties of the film. Although technologically relevant, such heteromolecular adsorbate systems have rarely been systematically investigated in the literature so far [32] , [33] , [34] , [35] , [36] , [37] , [38] , [39] , [40] , [41] , [42] , [43] , [44] , [45] . 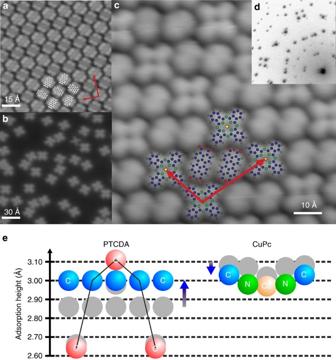Figure 1: Geometric structure of the MBW phase. (a–c) STM images of the homomolecular phases of (a) PTCDA/Ag(111), (b) CuPc/Ag(111) and (c) the MBW phase recorded at LHe temperature after room temperature deposition and at a sample bias ofUBias=−0.34, 0.34 and 0.20 V, respectively. The typical cross-like and elliptic shapes of CuPc and PTCDA molecules, respectively, are visible and illustrated by the atomic models superimposed in the figures. (d) Corresponding high-resolution LEED image indicating a commensurate structure. (e) Vertical adsorption geometry as revealed by NIXSW. The adsorption heights of all involved atomic species are illustrated for the MBW phase (coloured spheres) and the homomolecular adsorption systems (grey spheres). Figure 1: Geometric structure of the MBW phase. ( a – c ) STM images of the homomolecular phases of ( a ) PTCDA/Ag(111), ( b ) CuPc/Ag(111) and ( c ) the MBW phase recorded at LHe temperature after room temperature deposition and at a sample bias of U Bias =−0.34, 0.34 and 0.20 V, respectively. The typical cross-like and elliptic shapes of CuPc and PTCDA molecules, respectively, are visible and illustrated by the atomic models superimposed in the figures. ( d ) Corresponding high-resolution LEED image indicating a commensurate structure. ( e ) Vertical adsorption geometry as revealed by NIXSW. The adsorption heights of all involved atomic species are illustrated for the MBW phase (coloured spheres) and the homomolecular adsorption systems (grey spheres). Full size image As it turns out, at least three well-ordered mixed monolayer film structures with different CuPc/PTCDA stoichiometries exist on Ag(111). For the present investigation, we have selected a phase that contains one CuPc and two PTCDA molecules per unit cell and is commensurate with the Ag(111) surface; in the following, we refer to it as the mixed brick-wall (MBW) phase (see scanning tunnelling microscopy image and low-energy electron diffraction pattern shown in Fig. 1c,d , respectively). At first sight, both molecules retain their weak chemisorptive interaction with the substrate, but a closer look at adsorption heights and orbital binding energies reveal very interesting changes: in the MBW film the adsorption height for PTCDA (CuPc) is larger (smaller) than in the respective homomolecular films (see below and Fig. 1e ). Hence, the adsorption height suggests a weakening of the PTCDA–Ag and a strengthening of the CuPc–Ag bond. But the LUMO binding energies show a very different behaviour that breaks the normal relationship between adsorption height and orbital binding energies: we find that the PTCDA (CuPc) LUMO shifts to larger (smaller) binding energies, to the extent that the PTCDA LUMO becomes completely filled, while the CuPc LUMO is emptied; from the point of view of charge transfer, PTCDA is the winner who takes it all. Molecular adsorption heights In the following we analyse this remarkable situation in detail, first concentrating on the adsorption height. It can be measured with the highest precision (better than 0.05 Å) and chemical sensitivity by the NIXSW (normal incidence X-ray standing wave) technique. (For details regarding this and other experimental and computational methods see Supplementary Methods .) In Fig. 1e the vertical adsorption geometries are shown for all atomic species of the heteromolecular MBW phase (colour), and for the homomolecular monolayer structures (grey) [14] , [25] . All measured adsorption heights including their errors can be found in the Supplementary Table 1 . In both homomolecular phases (grey spheres) the molecules are distorted with respect to their planar geometries in the gas phase. The carboxylic oxygen atoms of PTCDA are closer to the surface than the perylene core due to the formation of a local Ag–O bonds [14] . However, with 2.86±0.01 Å the perylene core is still at a height significantly smaller than the sum of the van der Waals radii of the involved atomic species, which gives rise to a delocalized π-bond across the metal–organic interface and the significant charge transfer into the PTCDA LUMO, clearly seen with various spectroscopic techniques [21] , [46] , [47] . The distortion of CuPc is smaller and its overall adsorption distance is larger, indicating a weaker molecule–substrate interaction [25] . In the heteromolecular MBW phase (coloured spheres in Fig. 1e ) the perylene core of PTCDA is located significantly higher than that in the homomolecular phase, at 3.00±0.02 Å. According to the normal coupling between adsorption height and chemical interaction strength, this would indicate a weakening of the PTCDA–metal π-bond. For CuPc the situation is the opposite: its adsorption height becomes smaller on mixing with PTCDA (it changes from 3.08±0.02 to 3.04±0.02 Å), while its distortion is almost unchanged. Note that as a result of their mutual influence, both molecular backbones (and π-systems) adsorb approximately at the same height in the MBW phase. Electronic structure investigated by UPS The changes of interaction strength as inferred from geometry should be reflected in the electronic properties of the adsorbates, that is, in the energetic positions of the relevant frontier molecular orbitals [5] , [6] , [32] , [48] . 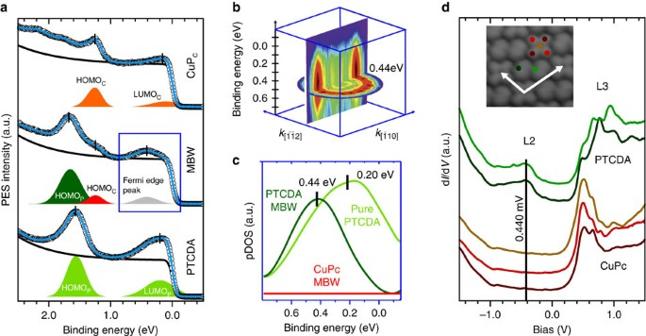Figure 2: Electronic structure of the MBW phase. (a) Conventional UPS data for homomolecular CuPc/Ag(111), the MBW and the homomolecular (herringbone) PTCDA/Ag(111) phase (from top to bottom). (b) Full tomographic 3D data cubeI(kx,ky,EB). An animated illustration is shown as Supplementary Movie 1 in the online version of the paper. (c) pDOS (resulting from the orbital tomography analysis) for the LUMOs of PTCDA and CuPc in the MBW phase as well as for the LUMO of PTCDA in its homomolecular phase. (d) Scanning tunnelling spectra recorded at five different positions, which are marked and colour coded in the STM image shown as inset. Figure 2a shows the valence band structure of the MBW film and both homomolecular structures, recorded by conventional ultraviolet photoelectron spectroscopy (UPS). For both homomolecular films, two features are visible: the peaks at higher binding energies correspond to the respective highest occupied molecular orbitals (HOMOs) and those in the vicinity of the Fermi level represent the former LUMOs and are visible in photoelectron spectroscopy only because they become partially filled due to charge transfer from the substrate and shift below the Fermi edge [21] , [25] , [47] . The partially filled LUMOs are an unambiguous proof for the chemisorptive interaction in both homomolecular films. For the heteromolecular structure one might naively expect a superposition of these two spectra, which is correct regarding the HOMO region. Both HOMO peaks are only slightly shifted compared with the homomolecular phases. However, for the LUMO levels close to the Fermi edge the situation is different: only one peak is visible at a significantly larger binding energy compared with both homomolecular films. Whether this ‘Fermi edge peak’ corresponds to the LUMO of PTCDA or CuPc or both cannot be judged from the spectrum shown in Fig. 2a . However, in any case, since it is not cut by the Fermi level, it corresponds to molecular orbital(s) that is/are completely occupied. Figure 2: Electronic structure of the MBW phase. ( a ) Conventional UPS data for homomolecular CuPc/Ag(111), the MBW and the homomolecular (herringbone) PTCDA/Ag(111) phase (from top to bottom). ( b ) Full tomographic 3D data cube I ( k x , k y , E B ). An animated illustration is shown as Supplementary Movie 1 in the online version of the paper. ( c ) pDOS (resulting from the orbital tomography analysis) for the LUMOs of PTCDA and CuPc in the MBW phase as well as for the LUMO of PTCDA in its homomolecular phase. ( d ) Scanning tunnelling spectra recorded at five different positions, which are marked and colour coded in the STM image shown as inset. Full size image Electronic structure as revealed by ARPES orbital tomography More insight in the origin of the Fermi edge peak can be gained from molecular orbital tomography, a recently developed analysis method for ARUPS data [21] , [49] . In orbital tomography, the angular distribution of photoelectrons is used as a k -space fingerprint of the emitting molecular orbital, allowing its identification by its symmetry and spatial probability distribution. Measuring a k -resolved data cube of photoelectron intensities in the binding energy range of the Fermi edge peak ( Fig. 2b and Supplementary Movie 1 ) and deconvoluting it in k -space into a superposition of momentum maps from all orbitals that could possibly contribute, we obtain the orbital-specific experimental projected densities of states (pDOS) displayed in Fig. 2c . In addition to the LUMOs of CuPc and PTCDA in the heteromolecular MBW phase, we also included the LUMO of PTCDA in the homomolecular phase, which is discernible from the MBW-PTCDA LUMO due to different in-plane orientations of the molecules. This parasitic contribution had to be considered since homomolecular PTCDA and heteromolecular MBW phases coexisted on this sample (in contrast to other samples used for UPS and NIXSW data acquisition). A substrate contribution was also considered in the fit (not shown). For more details of the orbital tomography analysis of the ARPES data see Supplementary Fig. 1 . The results (see Fig. 2c ) are remarkable: apart from the contribution from the parasitic homomolecular PTCDA islands (light-green curve), only one contribution is non-zero, namely, that for PTCDA in the MBW geometry (dark-green curve). It shows a maximum at E B =0.44 eV, matching the peak position of the conventional UPS experiment ( Fig. 2a ). The pDOS of CuPc (red curve), however, vanishes completely in the entire relevant binding energy region. This clearly demonstrates that the Fermi edge peak stems exclusively from the PTCDA LUMO. Also, the LUMO binding energy of PTCDA has increased in the MBW phase, leading to an enhanced charge transfer from the substrate, which fills up the orbital completely. In contrast, the LUMO binding energy of CuPc has decreased, with the consequence that CuPc releases all of its acquired charge. Hence, the electronic signatures that normally go along with shorter bonding distances and thus stronger chemical interaction appear here in conjunction with larger bonding distances (for PTCDA), and vice versa for CuPc. Electronic structure confirmed by STS The results of our ARPES molecular tomography analysis are confirmed by STS (scanning tunnelling spectroscopy). This local technique gives direct access to the valence structure of individual molecules. In Fig. 2d , spectra recorded at five different positions that are characteristic for the geometric shapes of the CuPc and PTCDA LUMOs are plotted. For both PTCDA molecules in the unit cell, the LUMO resonance is detected at the binding energy of the Fermi edge peak (0.44 eV), while for all positions on the CuPc molecule the spectrum in the corresponding region is flat. Results of density functional theory Our experimental results regarding geometric and electronic structures appear paradoxical. We therefore turn to density functional theory (DFT), which has become very reliable for verifying and predicting adsorption heights and electronic energy levels for both homo- and heteromolecular adsorbate systems (see, for example, refs 1 , 6 , 42 , 43 , 44 and references therein). Here we employed a generalized gradient approximation for exchange-correlation effects [50] and an empirical van der Waals correction according to Grimme [51] . The calculations yield adsorption heights in good agreement with experiment, both for the homomolecular and the heteromolecular phases ( cf. Supplementary Table 1 ). Moreover, they confirm the frontier orbital binding energies and charging states of the CuPc and PTCDA LUMOs as determined by experiment. This can be seen in Fig. 3a where the pDOS of the MBW phase and of the homomolecular PTCDA/Ag(111) and CuPc/Ag(111) phases are displayed. The question thus arises: how can we understand the counterintuitive behaviour of geometric structure (adsorption heights) and electronic properties (LUMO binding energies) that is found in experiment and theory? 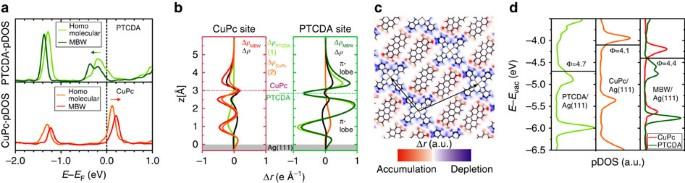Figure 3: Electronic structure as revealed by DFT. (a) Spin-up pDOS of the π-orbitals of PTCDA (upper panel) and CuPc (lower panel) in their homo- and heteromolecular phases, respectively. The spin-down pDOS is shown in theSupplementary Fig. 2. (b) Charge density reorganization Δρ, horizontally integrated in the adsorption site area, for CuPc (left panel) and PTCDA (right panel), plotted versus the distance to the surface (molecular planes atz≈3.0 Å). (c) Charge density difference plot showing depletion (blue) and accumulation (red) of electronic charge in a plane parallel to the surface 0.5 Å above the molecular plane (in a height of maximum DOS of the LUMO orbitals). (d) pDOS of the π orbitals of PTCDA and CuPc in the homomolecular PTCDA/Ag(111) (left), the homomolecular CuPc/Ag(111) (middle) and the heteromolecular MBW phase (right). Energies are aligned with the vacuum level, the Fermi energies are indicated by black lines revealing the work functions. Figure 3: Electronic structure as revealed by DFT. ( a ) Spin-up pDOS of the π-orbitals of PTCDA (upper panel) and CuPc (lower panel) in their homo- and heteromolecular phases, respectively. The spin-down pDOS is shown in the Supplementary Fig. 2 . ( b ) Charge density reorganization Δ ρ , horizontally integrated in the adsorption site area, for CuPc (left panel) and PTCDA (right panel), plotted versus the distance to the surface (molecular planes at z ≈3.0 Å). ( c ) Charge density difference plot showing depletion (blue) and accumulation (red) of electronic charge in a plane parallel to the surface 0.5 Å above the molecular plane (in a height of maximum DOS of the LUMO orbitals). ( d ) pDOS of the π orbitals of PTCDA and CuPc in the homomolecular PTCDA/Ag(111) (left), the homomolecular CuPc/Ag(111) (middle) and the heteromolecular MBW phase (right). Energies are aligned with the vacuum level, the Fermi energies are indicated by black lines revealing the work functions. Full size image On the way to a cogent model of the heteromolecular phase, we first turn to the remarkable fact that in the MBW phase PTCDA and CuPc equalize their adsorption heights. To first order, the adsorption height of a molecule on a metal is determined by the contact distance between the molecular backbone and the electron density that spills out from the surface. Hybridization with molecular orbitals, charge transfer and the so-called push-back effect will modify the charge profile above the bare surface. This reorganization is material specific, and depends on the chemical character of the molecule and the balance between chemisorption and physisorption for the given interface. But once these changes have been effected, the adsorbate essentially floats in contact on this rearranged electron density profile. This state of affairs precludes strongly dissimilar adsorption heights of neighboring molecules, since it is energetically unfavourable either to have a laterally structured evanescent metallic electron density or to have one of the molecular species sinking too deep into the laterally averaged electron spill out (PTCDA) or hovering too far above it (CuPc). Therefore, we must expect an equalization of the adsorption heights if the two molecules are laterally intermixed on a molecular length scale. But why are the adsorption heights of CuPc and PTCDA in their homomolecular phases different in the first place? Looking at the work function changes that both molecules effect on the surface, we observe that PTCDA increases the bare work function of Ag(111) to 4.76±0.02 eV, while CuPc reduces it to 4.15±0.02 eV. Note that all numbers given here are valid for closed monolayer films. Our DFT calculation, which reproduces these experimental values with great accuracy ( cf. Supplementary Table 2 ), allows an analysis of these changes: the work function change has two contributions, the bond dipole that arises from the charge reorganization and transfer on adsorption, and the bending dipole that stems from the adsorption-induced molecular distortion. It turns out that in the case of PTCDA/Ag(111) the charge transfer from the metal to the molecule is dominant, it contributes +0.50 eV to the work function change. For CuPc/Ag(111), it is the push-back effect that contributes most strongly with −0.55 eV. These numbers (note the opposite signs) reveal the different character of PTCDA and CuPc when they adsorb on Ag(111): the chemical component (charge transfer) of the bonding with Ag(111) is more prominent for PTCDA than it is for CuPc, while the reverse is true for the physisorptive contribution (push-back). This is the origin of the different adsorption heights: PTCDA pulls charge from the evanescent electron density into its LUMO and can therefore approach the surface more closely, while CuPc mainly pushes the evanescent electron density back into the metal, which precludes a closer approach, even though a (smaller) charge transfer from Ag(111) to CuPc is observed as well (see above) [3] , [25] . Figure 3b reveals the reorganization of the charge density that goes along with the equalization of adsorption heights on formation of the MBW phase. We have, separately for each type of molecule in the MBW phase, integrated the electron density reorganization Δ ρ MBW in the horizontal plane over the area of the respective molecules and plotted their z -dependence (red and dark-green lines). For comparison we have calculated the analogous quantities for two reference structures, namely (1) PTCDA molecules in the MBW unit cell from which CuPc has been removed (Δ ρ PTCDA , light-green line shown in Fig. 3b) and (2) CuPc molecules in the MBW unit cell from which PTCDA has been removed (Δ ρ CuPc , orange line). The differences of these electron density reorganization profiles, Δ ρ =Δ ρ MBW −(Δ ρ CuPc +Δ ρ PTCDA ), are plotted as black curves (for more details see Supplementary Fig. 3 ). The electron depletion of the CuPc π-lobes (left panel, orange curve, at ≈2.5 and ≈3.5 Å) is a consequence of the push-back-dominated interaction of CuPc with Ag(111) (although a small charge transfer into the molecule is also visible at some z ), whereas the electron accumulation in the corresponding region of PTCDA (right panel, light-green line, at ≈2.2 and ≈3.4 Å) originates from charge transfer into its LUMO. Furthermore, the figure reveals two important facts: first, we observe that in reference structure (2), CuPc pushes electrons into the PTCDA vacancies (right panel, orange curve, shallow maximum at ≈1.0 Å), while in reference structure (1) PTCDA sucks up electrons from the CuPc vacancies (left panel, light-green curve, minimum at ≈1.0 Å). Second, once the vacancies are filled again by the corresponding molecules, the electron density surplus at the PTCDA site is redistributed and yields an increased electron density in the π-lobes of the PTCDA molecule (right panel, dark-green curve, the peaks at ≈2.2 and ≈3.4 Å are larger compared with the light-green curve), while the electron density deficiency at the CuPc site is redistributed to yield a reduced electron density in the π-lobes of CuPc (left panel, the minima in the red curve at ≈2.5 and ≈3.5 Å are deeper than in the orange curve). The charge accumulation and depletion at PTCDA and CuPc sites, respectively, also influences the interaction of the frontier orbitals with the metal states, since it manifests itself in a population/depopulation of the respective LUMOs, also illustrated by the lateral map shown in Fig. 3c , taken at z =3.5 Å. Note, however, that the electron densities also change directly above the substrate ( z ≈1 Å). This modifies the Pauli repulsion between the adsorbates and the metal and cancels the net attractive force acting on PTCDA in reference structure (1) as well as its net repulsive counterpart on CuPc in reference structure (2), and thus explains how the two molecules equalize their heights in the heteromolecular phase: the electronic charge that CuPc sheds from its LUMO and repels from its site is redirected towards PTCDA, with the result that PTCDA both floats on this ‘cushion’ of charge and accepts more of it into its LUMO, while CuPc sinks into the remaining ‘depression’ of the electron density. The necessity to equalize the heights of the two adsorbates thus harmonizes very well with the different chemical characters (relative donor versus relative acceptor) of the two molecules. Finally we want to understand the regulation of the mutual charge transfer between molecules and surface in context with the orbital alignments and work function. For the MBW/Ag(111) structure we have measured a work function of 4.44±0.02 eV. This is half way between the values for PTCDA/Ag(111) and CuPc/Ag(111) and in excellent agreement with the calculated work function of 4.40 eV. We revealed the latter value from calculated pDOS, which are plotted in Fig. 3d , for both hetero- and homomolecular systems with aligned vacuum levels. More importantly, this figure shows that the LUMOs of PTCDA and CuPc move away from the common Fermi level in opposite directions, owing to the work function averaging and the very different electron affinities of the molecules. The investigation of similar systems have revealed similar trends for core levels and filled valence levels (for example, the HOMO) [52] . In our case, the LUMO shift explains why in the heteromolecular phase the charge transfer into the PTCDA (CuPc) LUMO is larger (smaller) than in the respective homomolecular phases. Note that the different electron affinities of CuPc and PTCDA, which of course are an expression of their different chemical characters, change slightly on formation of the heteromolecular phase. In comparison with the respective homomolecular phases, the increase (decrease) of electronic charge transfer into PTCDA (CuPc) causes a more (less) negative charging of the molecule, and thereby reduces (increases) its electron affinity. To verify the role of the metal surface and its work function for the energy level alignment, we have carried out a computational control experiment: we calculated the level alignments for a free-standing MBW layer, that is, without surface. Compared with the full MBW/Ag(111) structure, we observe substantially smaller LUMO shifts (relative to the vacuum level, for details see Supplementary Fig. 4 ). This proves that the frontier orbital alignment observed on mixing the two species is caused by their interaction with the metal surface, not by direct intermolecular interactions. Furthermore, we find that the MBW phase is stabilized by 0.21 eV when charge reorganization between the PTCDA and CuPc sites (that is, surface-mediated charge transfer between the two molecules) is allowed, compared with a situation of direct intermolecular and separated molecule–substrate interaction only ( cf. Supplementary Table 3 ). Incidentally, the different chemical characters of the two adsorbates also explain why in the heteromolecular system island formation prevails (as opposed to the repulsive interaction observed for the homomolecular CuPc/Ag(111)): the opposite bond dipoles of PTCDA and CuPc attract each other, thus promoting the formation of a compact layer, even if the arrangement of molecules in the MBW phase is less amenable to the formation of a network of hydrogen bonds. The DFT calculation shows that the total bond dipole in the MBW phase is nearly zero (−0.02 eV), indicating a cancellation of the individual bond dipoles of CuPc and PTCDA. In conclusion, the electronic and geometric properties of the MBW phase emerge in the following way: if only CuPc is present on Ag(111), it will push the evanescent electron density back (not withstanding a small metal–molecule charge transfer), owing to its (compared with PTCDA) less electron-affine character; this limits its approach to the surface. If PTCDA is added, this charge repelled by CuPc, instead of being merely pushed back into the surface, is laterally redirected towards the electron-affine PTCDA. This charge reorganization, which leads to a tangible energy gain, has two consequences: first, the adsorption heights of CuPc and PTCDA nearly equalize, with PTCDA floating up and CuPc sinking in. This can be interpreted as a consequence of local work function changes: CuPc increases the local work function at the PTCDA site, while PTCDA reduces it at the CuPc site. Second, the global work function of the mixed interface acquires a value that is intermediate between CuPc/Ag(111) and PTCDA/Ag(111). This in turn controls the energy level alignment such that CuPc reduces its charge uptake from the surface, while PTCDA increases it. In other words, the two coadsorbates mutually amplify their natural chemical characters vis à vis Ag(111): in the vicinity of CuPc, PTCDA becomes a stronger acceptor, while in the vicinity of PTCDA, CuPc becomes even less of an acceptor, and—relative to PTCDA—turns into a donor. Since the chemical interaction of both molecules with the metallic states of the substrate is dominated by the LUMO, this means that the chemical component of the molecule–surface interaction is strengthened for PTCDA and weakened for CuPc. It is noteworthy that PTCDA both floats up on an electron density cushion and takes up negative charge. Similarly, CuPc sheds negative charge and sinks into an electron density depression. This breaks the normal relationship between adsorption height and LUMO binding energy. Ultimately, this breaking of the normal coupling can be traced back to the mutual amplification: in the heteromolecular case, it is the metal together with the respective partner molecule that determines the behaviour. The apparently paradoxical behaviour between geometric structure (adsorption height) and electronic properties (frontier orbital binding energy) of the heteromolecular MBW phase is resolved, and has thus revealed very clearly how observables such as vertical adsorption height, frontier orbital binding energies and charge transfer, for homomolecular as well heteromolecular systems, are linked and influence each other. The insight at this level has an obvious impact on the challenge of engineering the interfaces of heteromolecular materials for applications. How to cite this article: Stadtmüller, B. et al. Unexpected interplay of bonding height and energy level alignment at heteromolecular hybrid interfaces. Nat. Commun. 5:3685 doi: 10.1038/ncomms4685 (2014).